Tandem intercalation strategy for single-layer nanosheets as an effective alternative to conventional exfoliation processes Simple and effective generation of transition metal chalcogenides (TMCs) in a single-layer form has been a challenging task. Here we present a tandem molecular intercalation (TMI) as a new exfoliation concept for producing single-layer TMCs from multi-layer colloidal TMC nanostructures in solution phase. TMI requires tandem Lewis base intercalates, where short ‘initiator’ molecules first intercalate into TMCs to open up the interlayer gap, and the long ‘primary’ molecules then bring the gap to full width so that a random mixture of intercalates overcomes the interlayer force. Spontaneous exfoliation then yields single-layer TMCs. The TMI process is uniquely advantageous because it works in a simple one-step process under safe and mild conditions (that is, room temperature without sonication or H 2 generation). With the appropriate intercalates, we have successfully generated single-layer nanostructures of group IV (TiS 2 , ZrS 2 ), group V (NbS 2 ) and VI (WSe 2 , MoS 2 ) TMCs. Two-dimensional (2D) layered materials including transition metal chalcogenides (TMCs) with strong in-plane covalent bonds and weak interlayer van der Waals interactions exhibit a wide range of interesting anisotropic phenomena from charge transport to catalytic and optical properties [1] , [2] , [3] , [4] , [5] , [6] , [7] , [8] , [9] . Similar to graphene, such interesting effects are centred on single-layer TMCs and, as an example, when MoS 2 , an indirect band gap semiconductor in bulk, is thinned to a single layer, a strong photoluminescence is observed due to the indirect-to-direct band gap change [6] , [7] . Single-layer or few-layer nanosheets can be obtained from bulk TMCs by several exfoliation techniques such as dry mechanical cleavage with Scotch tape [10] , [11] or solution-based exfoliation processes [12] , [13] , [14] , [15] , [16] , [17] , [18] , [19] , [20] , [21] , [22] , [23] , [24] , [25] , [26] . Intercalation of alkali metals by using elemental metals [12] , [13] (for example, potassium) or organo-alkali compounds (for example, butyllithium [14] , [15] , [16] and more recently sodium naphthalenide [17] ) has been a widely used method for the exfoliation of layered materials. Such exfoliation and disintegration methods with K, air and EtOH-H 2 O along with sonication of layered flakes have successfully generated monolayer nanoparticles of WS 2 , BN and graphene [9] , [12] , [13] . Although quite effective, the use of reactive chemicals during exfoliation conditions and H 2 generation through multiple exfoliation processes has drawbacks [17] . While the electrochemical exfoliation method has been developed as a faster and controllable exfoliation protocol, complicated electrochemical set-ups present challenges for the mass production of single-layer nanosheets [18] , [19] , [20] , [21] . Alternatively, a sonication method in the presence of solvents [22] , [23] such as N -methyl-pyrrolidone has been demonstrated for the successful exfoliation of wide range of TMCs, but the products are often mixed with single- and multi-layer TMCs with potential degradation of samples due to the harsh sonication conditions required to overcome the interlayer interactions [24] , [25] , [26] . As stated here, current methodologies have their own advantages and disadvantages, but none of them are yet perfect [17] , [26] , although it is true that these are effective for large-size layered nanostructures. The development of mild exfoliation strategies that can circumvent the key harsh process conditions (for example, sonication and H 2 gas formation) has been challenging and, therefore, new and better routes to obtain single-layer TMCs in a simple, efficient and reproducible manner are currently being pursued. In this study, we introduce the ‘tandem molecular intercalation (TMI)’ process as a mild and effective exfoliation strategy for single-layer 2D TMC nanosheets from multi-layer colloidal TMC nanostuctures. Our TMI process utilizes two different Lewis base intercalates for the initiative and primary roles. Relatively short length ‘initiator’ Lewis base molecules are introduced into the interlayer space of 2D TMCs to start the gap-widening process, and a simultaneous influx of ‘primary’ intercalate molecules with longer chains creates randomly mixed bilayers of intercalates to overcome the interlayer interactions and eventually generate single-layer nanosheets ( Fig. 1 ). Although the host–guest chemistry for the intercalation of Lewis bases into bulk TMCs has been well documented [27] , [28] , its successful extension to an exfoliation strategy has not been demonstrated yet. 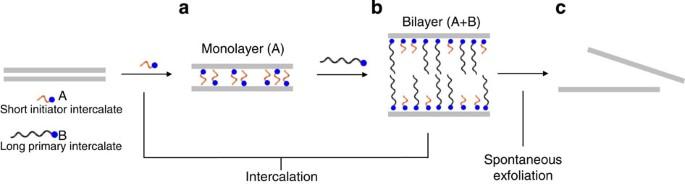Figure 1: Tandem molecular intercalation process for exfoliation of TMCs. The TMI process incorporates two different Lewis base intercalates. (a) Short ‘initiator’ intercalates (orange tail) are intercalated first into the interlayer gap, and (b) long ‘primary’ intercalates (black tail) then enter to form randomly mixed bilayers of intercalates and widen the interlayer gap. (c) Finally, TMCs with bilayer intercalates are spontaneously delaminated to single-layer nanosheets. Figure 1: Tandem molecular intercalation process for exfoliation of TMCs. The TMI process incorporates two different Lewis base intercalates. ( a ) Short ‘initiator’ intercalates (orange tail) are intercalated first into the interlayer gap, and ( b ) long ‘primary’ intercalates (black tail) then enter to form randomly mixed bilayers of intercalates and widen the interlayer gap. ( c ) Finally, TMCs with bilayer intercalates are spontaneously delaminated to single-layer nanosheets. Full size image Intercalation of alkylamine in TiS 2 colloidal nanostructure We first examined the group IV TiS 2 colloidal nanostructure (60 nm in diameter with a dozen layers) with an interlayer distance of 5.7 Å and with each single-layer TiS 2 comprising a S-Ti-S tri-atomic plate of 1T-type CdI 2 structure [29] ( Fig. 2a ). The intercalation and gap-widening capability of Lewis base molecular intercalates were investigated depending on the alkyl chain length of primary amines such as propyl-, butyl- and hexyl-amine ( Fig. 2b ) [29] , [30] . Here, an excess amount of intercalate is added to TiS 2 nanoparticle in dimethyl sulphoxide (DMSO) at room temperature, and the reaction mixture is stirred for 30 min to 5 h depending on the chain length of the intercalate molecules. Subsequently, the colloidal suspension is precipitated by centrifugation and washed with chloroform. The initial interlayer distance of pristine TiS 2 is 5.7 Å, but after intercalation with propyl- butyl- and hexyl-amine, it increases to 9.5, 10.5 and 14.3 Å, respectively, according to TEM analysis ( Fig. 2c–f ). 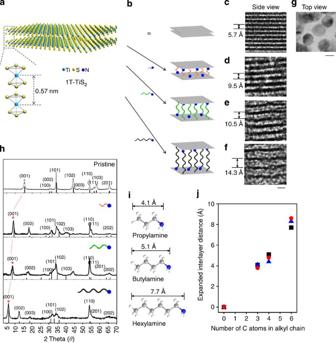Figure 2: Intercalate size-dependent interlayer expansion of multi-layer TiS2. (a) Visualization of TiS2using ball and stick model to illustrate the 2D layered structure. (b) Schematic illustration of interlayer distance change of TiS2by intercalating alkylamine. Side view of layers in TEM images (c) before intercalation and after intercalation of (d) propylamine, (e) butylamine and (f) hexylamine. Scale bar, 1 nm. (g) Top-view TEM image of multi-layer TiS2before exfoliation. Scale bar, 50 nm. (h) XRD patterns of pristine TiS2and intercalated TiS2with propylamine, butylamine and hexylamine. Vertical lines indicate reference peaks of bulk and expanded TiS2(JCPDS #15-0853). (i) Calculated length between nitrogen and terminal hydrogen of propylamine (4.1 Å), butylamine (5.1 Å) and hexylamine (7.7 Å) by ChemBio 3D® Ultra program. (j) Expanded interlayer distance of TiS2plotted against the number of carbon (C) atoms in alkyl chain of intercalate (black square, calculated value; blue triangle, value observed by XRD; red circle, value observed by TEM). Figure 2: Intercalate size-dependent interlayer expansion of multi-layer TiS 2 . ( a ) Visualization of TiS 2 using ball and stick model to illustrate the 2D layered structure. ( b ) Schematic illustration of interlayer distance change of TiS 2 by intercalating alkylamine. Side view of layers in TEM images ( c ) before intercalation and after intercalation of ( d ) propylamine, ( e ) butylamine and ( f ) hexylamine. Scale bar, 1 nm. ( g ) Top-view TEM image of multi-layer TiS 2 before exfoliation. Scale bar, 50 nm. ( h ) XRD patterns of pristine TiS 2 and intercalated TiS 2 with propylamine, butylamine and hexylamine. Vertical lines indicate reference peaks of bulk and expanded TiS 2 (JCPDS #15-0853). ( i ) Calculated length between nitrogen and terminal hydrogen of propylamine (4.1 Å), butylamine (5.1 Å) and hexylamine (7.7 Å) by ChemBio 3D® Ultra program. ( j ) Expanded interlayer distance of TiS 2 plotted against the number of carbon (C) atoms in alkyl chain of intercalate (black square, calculated value; blue triangle, value observed by XRD; red circle, value observed by TEM). Full size image XRD analysis also confirms the widening interlayer distance ( Fig. 2h ). Interlayer gap dependent c axis peaks, such as (001), (002) and (003), are shifted to lower angles as the intercalate size increases. Pronounced effects are observed for the (001) peak position, where the 2 θ angle changes from 15.5° to 9.0°, 8.7° and 6.3° for propylamine, butylamine and hexylamine, respectively. From the 2 θ values, the interlayer distances are calculated to be 5.7, 9.8, 10.2 and 14.0 Å, and the expansion of the c axis is 4.1 Å for propylamine, 4.5 Å for butylamine and 8.3 Å for hexylamine ( Fig. 2j ), respectively. This (001) peak shift trend and TEM analysis confirm that the interlayer gap widening of TiS 2 is proportional to the alkylamine length. As the lengths of propyl-, butyl- and hexyl-amine are ~4.1, 5.1 and 7.7 Å ( Fig. 2i ), respectively, the observed expansion of the interlayer gap suggests a head-to-tail monolayer arrangement of alkylamines between the layers [31] . This alkylamine intercalation process proceeds through a monolayer arrangement at the initial stage, but after lengthened intercalation time, the intercalates start to adopt a bilayer arrangement between the layers. With the use of propylamine, the 2 θ angle of the (001) peak position of TiS 2 shifts from 15.5° to 8.9° at 45 min and 6.4° at 7 h ( Fig. 3a ). At the intermediate time of 3 h, the two peaks at 8.9° and 6.4° are simultaneously observed. These XRD results suggest that the TiS 2 interlayer distance of 9.9 Å corresponds to a monolayer of propylamine, which subsequently changes to a bilayer formation (13.8 Å) through an intermediate state (3 h) ( Fig. 3b ). The intercalation modes of alkylamines follow monolayer to bilayer arrangements, and the interlayer gap widening can be controlled using different alkylamine intercalates. However, none of the layered TiS 2 show spontaneous exfoliation even though the London-dispersion-corrected DFT calculation estimates a critical interlayer distance of ~11 Å to overcome the interlayer van der Waals interaction between two layers of pristine TiS 2 ( Fig. 3c ). Our observation of non-exfoliation phenomenon is presumably due to the additional energy needed to overcome partially or fully interdigitated interactions between the alkyl chains of the intercalates ( Fig. 3b ) [30] , [32] , [33] . 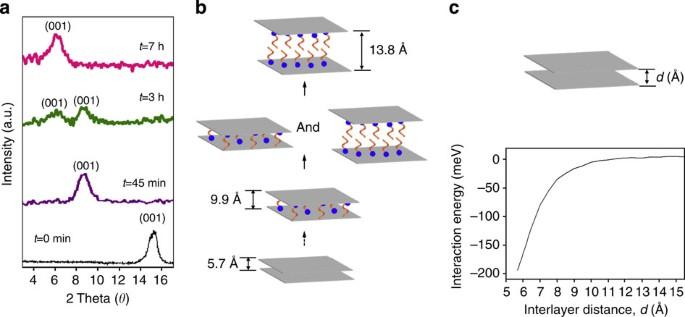Figure 3: Time-dependent interlayer distance change of multi-layer TiS2with propylamine. (a) XRD patterns of intercalated TiS2at 0 min, 45 min, 3 h and 7 h after treatment of propylamine. (b) Illustration of interlayer distance change of TiS2by intercalating propylamine. (c) Interlayer interaction energy calculated by density functional theory at the PBE-D3-BJ level. The critical interlayer distance for pristine TiS2exfoliation is estimated to be ~11.0 Å, where the interaction energy is close to ~kBT. Figure 3: Time-dependent interlayer distance change of multi-layer TiS 2 with propylamine. ( a ) XRD patterns of intercalated TiS 2 at 0 min, 45 min, 3 h and 7 h after treatment of propylamine. ( b ) Illustration of interlayer distance change of TiS 2 by intercalating propylamine. ( c ) Interlayer interaction energy calculated by density functional theory at the PBE-D3-BJ level. The critical interlayer distance for pristine TiS 2 exfoliation is estimated to be ~11.0 Å, where the interaction energy is close to ~ k B T. Full size image Exfoliation of TMCs via TMI method Here, we devised the TMI concept, where two different lengths of intercalates are utilized for the exfoliation of layered nanostructures. This TMI process has distinctive features, namely a short ‘initiator’ alkylamine first expands the interlayer gap for efficient intercalation of the ‘primary’ long alkylamine; the difference in the chain length, then, generates a bilayer arrangement with empty space between intercalates to reduce van der Waals force between them; and finally spontaneous exfoliation occurs ( Fig. 4a ). We examined the TMI concept for the exfoliation of multi-layer TiS 2 . By adding propylamine and hexylamine to colloidal TiS 2 nanostructure in DMSO at room temperature, the intercalation of propylamine is observed with an expanded interlayer distance of 9.5 Å in 30 min ( Fig. 4b ), and the presence of intercalated propylamine is confirmed by 1 H-NMR. Then, further expansion of the layer distance to 21 Å is observed in 6 h ( Fig. 4c ), and the coexistence of propylamine and hexylamine is confirmed by 1 H-NMR. At this stage, the layers spontaneously begin to separate, and single-layer TiS 2 nanosheets are obtained. 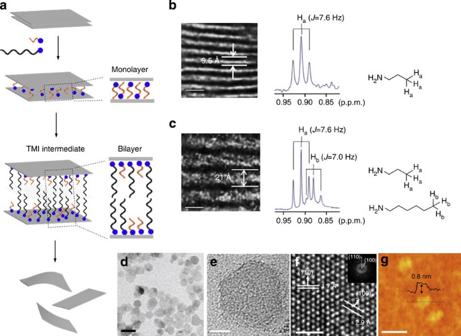Figure 4: Exfoliation of multi-layer TiS2nanostructure by TMI process. (a) Illustration of tandem molecular intercalates (TMI) process. Side-view TEM image and1H-NMR spectrum of TiS2intercalated with (b) propylamine and (c) both propylamine and hexylamine. (d) Top-view and (e) magnified TEM images of TiS2after exfoliation. (f) HRTEM image and FFT pattern (inset) of a single-layer TiS2nanosheet. (g) AFM image of single-layer TiS2nanosheets. Scale bars, 2 nm inbandc; 100 nm indandg; 20 nm ine; 1 nm inf. Figure 4d,e show TEM images of single-layer TiS 2 nanosheets after exfoliation. A top-view high-resolution TEM (HRTEM) image of a single-layer TiS 2 nanosheet shows lattice fringes with interplanar spacings of 2.9 and 1.7 Å, corresponding to the (100) and (110) planes of the TiS 2 , respectively ( Fig. 4f ). The single-layer thickness of 8.0 Å is confirmed by AFM analysis ( Fig. 4g ). Additional XRD analysis shows single peak of (110) plane at 53.7° without any peaks in c axis direction, which confirms that final products are fully exfoliated single-layer TiS 2 ( Supplementary Figs 1a and 2b ). Such experimental observations are in good agreement with the calculations based on density-functional tight-binding theory, which confirms that mixed intercalates of different chain lengths decrease the total interaction energy below 2 k B T to have an effective exfoliation ( Supplementary Fig. 3 , Supplementary Tables 1–3 ). Figure 4: Exfoliation of multi-layer TiS 2 nanostructure by TMI process. ( a ) Illustration of tandem molecular intercalates (TMI) process. Side-view TEM image and 1 H-NMR spectrum of TiS 2 intercalated with ( b ) propylamine and ( c ) both propylamine and hexylamine. ( d ) Top-view and ( e ) magnified TEM images of TiS 2 after exfoliation. ( f ) HRTEM image and FFT pattern (inset) of a single-layer TiS 2 nanosheet. ( g ) AFM image of single-layer TiS 2 nanosheets. Scale bars, 2 nm in b and c ; 100 nm in d and g ; 20 nm in e ; 1 nm in f . Full size image Our tandem molecular exfoliation method can be applied to other colloidal nanoparticles of group IV, V and VI TMCs, such as ZrS 2 , NbS 2 and WSe 2 . First, the exfoliation of multi-layer ZrS 2 nanostructure (17 nm in lateral size and three layers) is examined ( Fig. 5a,b ). Although less explored than group VI counterparts, group IV TMCs also exhibit interesting single-layer properties such as enhanced thermoelectric property and electrical conductivity for TiS 2 and strain-driven indirect-to-direct band gap transition of ZrS 2 (refs 34 , 35 , 36 ). Similar to the case of TiS 2 , propylamine and hexylamine are added to ZrS 2 nanostructure in DMSO with stirring at room temperature. After 4 h, the interlayer distance is expanded from 5.8 Å ( Fig. 5b ) to 20.5 Å ( Fig. 5c ). After 9 h, single-layer ZrS 2 nanosheets are obtained after centrifugation ( Fig. 5d ). The thickness measured by TEM is ~6.0 Å, which is consistent with the estimated thickness of single-layer ZrS 2 ( Fig. 5e ). A top-view HRTEM image of a single-layer ZrS 2 nanosheet shows lattice fringes with interplanar spacings of 3.1 and 1.8 Å, corresponding to the (100) and (110) planes of the hexagonal 1T-ZrS 2 , respectively ( Fig. 5f and Supplementary Fig. 2c ). This TMI method with propyl- and hexylamine intercalates is also effective to group V NbS 2 nanoparticles ( Supplementary Fig. 4 ). 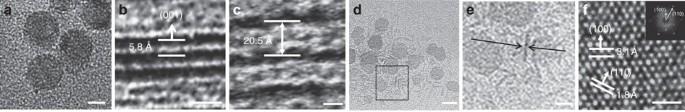Figure 5: Exfoliation of multi-layer ZrS2nanostructure. (a) Top-view and (b) side-view TEM image of three-layer ZrS2nanostructure before exfoliation. (c) Side-view TEM image of propylamine and hexylamine intercalated ZrS2. (d) TEM image and (e) magnified TEM image of the single-layer ZrS2nanosheets in the box ofd. A side-view of the single-layer ZrS2nanosheet between the arrows. (f) HRTEM image and FFT pattern (inset) of a single-layer ZrS2nanosheet. Scale bars, 10 nm inaande; 1 nm inb,candf; 20 nm ind. Figure 5: Exfoliation of multi-layer ZrS 2 nanostructure. ( a ) Top-view and ( b ) side-view TEM image of three-layer ZrS 2 nanostructure before exfoliation. ( c ) Side-view TEM image of propylamine and hexylamine intercalated ZrS 2 . ( d ) TEM image and ( e ) magnified TEM image of the single-layer ZrS 2 nanosheets in the box of d . A side-view of the single-layer ZrS 2 nanosheet between the arrows. ( f ) HRTEM image and FFT pattern (inset) of a single-layer ZrS 2 nanosheet. Scale bars, 10 nm in a and e ; 1 nm in b , c and f ; 20 nm in d . Full size image For the exfoliation of multi-layer WSe 2 nanostructure, tandem intercalates with high Lewis basicity are chosen. Two different-length intercalates of sodium ethoxide and sodium hexanolate are added to multi-layer WSe 2 nanostructure in DMSO. After stirring for 7 h at room temperature, single-layer WSe 2 nanosheets are isolated by centrifugation. During the course of intercalation, the expansion of the 6.5 Å interlayer spacing of WSe 2 ( Fig. 6g ) to 12.2 Å ( Fig. 6h ) suggests that ethoxide intercalation proceeds to form a bilayer arrangement between the layers. 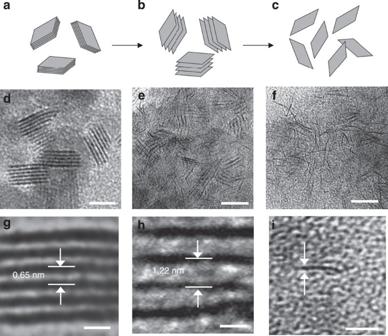Figure 6: Exfoliation of multi-layer WSe2nanostructure. (a–c) Schematic illustration of WSe2exfoliation processes. (d–f) Low-magnification and (g–i) magnified side-view TEM image of starting multi-layer WSe2nanostructures (d,g), WSe2intercalated with ethoxide in bilayer arrangement (e,h) and single-layer WSe2nanosheets (f,i). Scale bars, 5 nm indandi; 10 nm ineandf; 1 nm ingandh. Figure 6f,i show low-magnification and magnified TEM images of single-layer WSe 2 nanosheets after exfoliation, where a side view of standing single-layer WSe 2 nanosheets is observed. This exfoliation process can be scaled up to sub-gram scale ( Supplementary Fig. 5 ). Figure 6: Exfoliation of multi-layer WSe 2 nanostructure. ( a – c ) Schematic illustration of WSe 2 exfoliation processes. ( d – f ) Low-magnification and ( g – i ) magnified side-view TEM image of starting multi-layer WSe 2 nanostructures ( d , g ), WSe 2 intercalated with ethoxide in bilayer arrangement ( e , h ) and single-layer WSe 2 nanosheets ( f , i ). Scale bars, 5 nm in d and i ; 10 nm in e and f ; 1 nm in g and h . Full size image The choice of proper intercalates is critical to have their effective intercalation into TMCs. Intercalates act as Lewis base with highest occupied molecular orbital (HOMO) and TMCs act as Lewis acid with lowest unoccupied molecular orbital (LUMO). Therefore, as the HOMO–LUMO energy difference (ΔE HOMO–LUMO ) is smaller, the more favoured their interaction becomes. Such HOMO–LUMO Lewis acid–base interaction can be generally applied to group IV and VI TMCs. LUMO of group VI TMCs (for example, MoS 2 , MoSe 2 , MoTe 2 , WS 2 , WSe 2 and WTe 2 ) is between −4.2 and −3.5 eV, which is in close energy level with HOMO (approximately −4.2 eV) of strong base alkoxides to have favoured interactions between them [37] , [38] . Similarly, LUMO of group IV TMCs (for example, TiS 2 , ZrS 2 , ZrSe 2 , HfS 2 and HfSe 2 ) is ranging from −6.0 to −5.5 eV, which is close to HOMO (approximately −6.2 eV) of relatively weaker base alkylamines [37] , [38] , [39] . While our TMI method is most effective for the exfoliation of laterally small (<100 nm) TMC nanoparticles, it can be also extended to larger micron-size TMCs. For the exfoliation of micron-size TMCs ( Fig. 7 and Supplementary Fig. 6 ), sodium ethoxide and hexanolate are added to a solution of MoS 2 in DMSO. After stirring 48 h, single-layer MoS 2 nanosheets over 1 μm are observed ( Fig. 7 ). Similarly, micron-size multi-layer TMCs of WSe 2 and TiS 2 can also be exfoliated ( Supplementary Figs 2a and 6 ). Although specific conditions (for example, time, type and concentration of intercalates, temperature and so on) should be further optimized for efficient exfoliation, this preliminary study indicates the potential of TMI method for large-size TMCs. 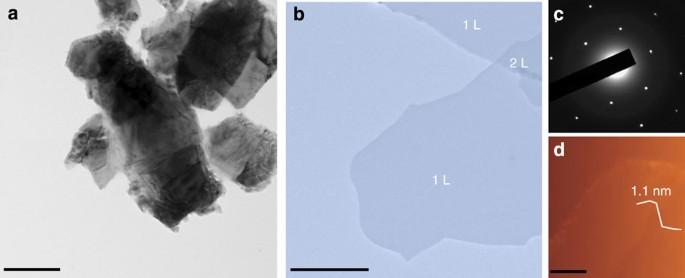Figure 7: Micron-size MoS2exfoliation by TMI method. (a) TEM image of micron size multi-layer MoS2. (b) TEM image (pseudo-colour) of exfoliated single-layer MoS2(L, layer). (c) SAED pattern and (d) AFM image of exfoliated MoS2. Scale bars, 1 μm ina; 0.5 μm inb; 0.1 μm ind. Figure 7: Micron-size MoS 2 exfoliation by TMI method. ( a ) TEM image of micron size multi-layer MoS 2 . ( b ) TEM image (pseudo-colour) of exfoliated single-layer MoS 2 (L, layer). ( c ) SAED pattern and ( d ) AFM image of exfoliated MoS 2 . Scale bars, 1 μm in a ; 0.5 μm in b ; 0.1 μm in d . Full size image In this study, we demonstrate that ‘tandem molecular intercalation (TMI)’ is an effective new concept for the exfoliation of multi-layer colloidal TMC nanostructures into single-layer TMC nanosheets. TMI is a relatively fast process for producing single-layer TMCs and is conducted at room temperature, with the clear merit of eliminating the occasional degradation of single-layer TMCs by avoiding harsh exfoliation processes. A variety of Lewis bases can be intercalated into TMC nanostructures, and group IV (TiS 2 and ZrS 2 ), group V (NbS 2 ) and VI (WSe 2 , MoS 2 ) TMCs require different types of intercalates. A relatively weaker Lewis base, such as alklyamine, works nicely for group IV and V TMCs, whereas a stronger Lewis base, such as alkoxide, is required for group VI TMCs. In principle, TMI can serve as a general strategy for the exfoliation of wide range of colloidal TMC nanostructures under mild exfoliation conditions, namely, a room-temperature process without sonication or H 2 evolution. Alkylamine chain length-dependent intercalation Propylamine (0.07 ml, 0.91 mmol), pre-synthesized TiS 2 (ref. 40 ; 0.05 mmol) and DMSO (5 ml) are added to a 10 ml vial. The mixture is stirred for 30 min at room temperature. The mixture is then precipitated by centrifugation at 3,000 r.p.m. for 30 min, and the precipitates are washed three times with chloroform. The intercalation conditions for other alkylamines are identical except for the intercalation time (1 h for butylamine and 5 h for hexylamine). Exfoliation of multi-layer TMC nanostructures Multi-layer colloidal TiS 2 nanostructure (5.0 mg, 0.04 mmol) [40] , propylamine (3.0 ml, 36.5 mmol), hexylamine (2.0 ml, 15.1 mmol) and DMSO (5 ml) are mixed to a 10 ml vial and stirred for 10 h at room temperature. Then, the mixture is centrifuged at 3,000 r.p.m. for 30 min to precipitate non-exfoliated materials. The supernatant is re-centrifuged at 15,000 r.p.m. for 50 min to precipitate exfoliated TMCs. Then, chloroform (10 ml) is added to dissolve the precipitate and the resulting purple solution is centrifuged at 17,500 r.p.m. for 10 min. This process repeats several times and then the final product is dried under vacuum at room temperature for 2 h to afford exfoliated TiS 2 (1.4 mg, 27%) as a purple powder. The exfoliation of multi-layer ZrS 2 follows similar procedures. Multi-layer colloidal ZrS 2 nanostructure (5.0 mg, 0.03 mmol) [40] , propylamine (2.5 ml, 30.4 mmol), hexylamine (1.0 ml, 7.6 mmol) and DMSO (5 ml) are mixed to a 10 ml vial and stirred for 9 h at room temperature. Single-layer ZrS 2 (1.6 mg, 32%) is obtained by following the same purification process of TiS 2 . For the exfoliation of WSe 2 , multi-layer colloidal WSe 2 nanostructure (10.0 mg, 0.03 mmol), sodium ethoxide (1.50 g, 22.0 mmol), sodium hexanolate (0.50 g, 4.03 mmol) and DMSO (15 ml) are mixed. After 7 h stirring, the mixture is centrifuged at 6,000 r.p.m. for 30 min to precipitate the non-exfoliated materials. Then the supernatant is re-centrifuged at 15,000 r.p.m. for 60 min to precipitate exfoliated TMCs. The precipitate is washed several times with ethanol via centrifugation at 17,500 r.p.m. for 20 min to give exfoliated WSe 2 (3.3 mg, 33%). Instruments TEM and HRTEM analyses were performed using JEM 2100 at 200 kV and JEOL-ARM1300S at 1,250 kV, respectively. Atomic force microscopy (AFM) images were obtained in non-contact mode using a scanning probe microscope (Veeco). X-ray diffraction (XRD) studies were conducted using Rigaku-G2005304 equipped with a Cu kα radiation source (30 kV, 15 mA). 1 H-NMR spectra were obtained using a 400 MHz FT-NMR Spectrometer (Bruker Biospin). Density-functional theory calculations The DFT calculations were performed using the Amsterdam Density-Functional (ADF2013-BAND) package [41] , [42] . We used the local VWN exchange-correlation potential with nonlocal Perdew–Burke–Ernzerhof exchange-correlation correction and empirical D3 treatment of London dispersion interactions (PBE-D3-BJ) [43] . How to cite this article : Jeong, S. et al. Tandem intercalation strategy for single-layer nanosheets as an effective alternative to conventional exfoliation processes. Nat. Commun. 6:5763 doi: 10.1038/ncomms6763 (2015).